Abundance of live244Pu in deep-sea reservoirs on Earth points to rarity of actinide nucleosynthesis Half of the heavy elements including all actinides are produced in r -process nucleosynthesis, whose sites and history remain a mystery. If continuously produced, the Interstellar Medium is expected to build-up a quasi-steady state of abundances of short-lived nuclides (with half-lives ≤100 My), including actinides produced in r -process nucleosynthesis. Their existence in today’s interstellar medium would serve as a radioactive clock and would establish that their production was recent. In particular 244 Pu, a radioactive actinide nuclide (half-life=81 My), can place strong constraints on recent r -process frequency and production yield. Here we report the detection of live interstellar 244 Pu, archived in Earth’s deep-sea floor during the last 25 My, at abundances lower than expected from continuous production in the Galaxy by about 2 orders of magnitude. This large discrepancy may signal a rarity of actinide r -process nucleosynthesis sites, compatible with neutron-star mergers or with a small subset of actinide-producing supernovae. About half of all nuclides existing in nature and heavier than iron are generated in stellar explosive environments. Their production requires a very short and intense burst of neutrons (rapid neutron capture or r -process) [1] , [2] , [3] . The nuclides are formed via successive neutron captures on seed elements, following a path in the very neutron-rich region of nuclei. However, the relevant astrophysical sites, with supernovae (SN) [1] , [2] and neutron-star (NS-NS) mergers [3] , [4] as prime candidates, and the history of the r -process during the Galactic chemical evolution are largely unknown. The interstellar medium (ISM) is expected to become steadily enriched with fresh nucleosynthetic products and may also contain continuously produced short-lived nuclides (with half-lives ≤100 My (ref. 5 )), including actinides produced in r -process nucleosynthesis. Recent r -process models within SNe-II explosions, based on neutrino wind scenarios [6] , [7] , suffer difficulties on whether heavy elements can really be produced in these explosions. An alternative site is NS ejecta, for example, NS-NS or NS black-hole (NS-BH) mergers. Candidates of such neutron-star binary systems have been detected [8] , [9] . Estimations of an NS-NS merger event rate of about (2–3) × 10 −5 per year in our galaxy would allow for such mergers to account for all heavy r -process matter in our Galaxy [3] , [10] , [11] . It was pointed out by Thielemann et al . [4] that observations of old stars indicate a probable splitting of the r -process into (i) a rare event that reproduces the heavy r -process abundances including actinides always in solar proportions, and (ii) a more frequent event responsible for the lighter r -process abundances. Galactic chemical evolution models [10] , [12] , [13] show that NS mergers, occurring at late time in the life of a galaxy, cannot account for all the r -process nuclei found in very old stars [12] . Thus, recent models suggest different r -process scenarios (similar to s process), which might occur at different nucleosynthesis sites [3] , [13] . To summarize, very few hints on astrophysical sites and galactic chemical evolution exist. First, the relative abundance distribution observed spectroscopically in a few old stars for r -process elements between barium and hafnium is very similar to that of the Solar System (SS) [1] , [14] , pointing to an apparently robust phenomenon; a large scatter for the r -process elements beyond Hf and also below barium is, however, observed [3] , [11] , [15] . Second, the early SS (ESS) is known to have hosted a set of short-lived radioactive nuclides ( t 1/2 <~100 My) [5] , [16] , [17] , [18] , among them pure r -process nuclei such as 244 Pu (half-life=81 My) and 247 Cm (15.6 My) clearly produced no more than a few half-lives before the gravitational collapse of the protosolar nebula [19] , [20] , [21] , [22] , [23] . We report here on a search for live 244 Pu (whose abundance in the ESS relative to 238 U was ~0.8% (see refs 5 , 19 , 20 , 21 , 23 , 24 , 25 )) in deep-sea reservoirs, which are expected to accumulate ISM dust particles over long time periods. Our findings indicate that SNe, at their standard rate of ~1–2/100 years in the Galaxy, did not contribute significantly to actinide nucleosynthesis for the past few hundred million years. A similar conclusion is drawn, when related to the recent SNe history in the local interstellar environment: we do not find evidence for live 244 Pu that may be locked in the ISM in accumulated swept-up material and that was transported to Earth by means of recent SNe activity. Our results suggest that actinide nucleosynthesis, as mapped through live 244 Pu, seems to be very rare. Experimental concept ISM dust particles [26] , [27] , assumed to be representative of the ISM, are known to enter the SS and are expected to reach and accumulate on Earth in long-term natural depositories such as deep-sea hydrogenous iron-manganese (FeMn) encrustations and sediments. Such a process is confirmed by inclusion in these archives of meteoritic 10 Be, cosmogenic 53 Mn and live 60 Fe, the latter attributed to the direct ejecta of a close-by SN (refs 28 , 29 , 30 ). 244 Pu-detection would be the equivalent for r -process nuclides of the γ-ray astronomy observations of live radioactivities [17] produced by explosive nucleosynthesis in single SN events (for example, 56 Ni (6.1 d), 56 Co (77.3 d), 44 Ti (60.0 y) or diffuse in the Galactic plane such as 26 Al (0.72 My) and 60 Fe (2.62 My), owing to their longer half-life). Several models, based on the frequency of SN events, the nucleosynthesis yield and the radioactive half-life, were developed to calculate the abundance of 244 Pu in quasi-secular equilibrium between production and radioactive decay rates. These models together with the flux and average mass of ISM dust particles into the inner SS measured by space missions in the last decade (Galileo, Ulysses, Cassini) [31] are used here to estimate the corresponding influx of 244 Pu nuclei onto Earth. We compare our results also with a possible imprint of recent actinide nucleosynthesis (<15 My) from the SNe history of the Local Bubble (LB, a cavity of low density and hot temperature of ~200 pc diameter). Recent ISM simulations suggest about 14–20 SN explosions within the last 14 My [32] , [33] , [34] that were responsible for forming the local ISM structure and the LB. 244 Pu decay can be considered negligible during this period. The SN ejecta shaped the ISM and also accumulates swept-up material including pre-existing 244 Pu from nucleosynthesis events prior to the formation of the LB [35] , [36] . With a growth rate of a few millimetres per million years [37] , hydrogenous crusts will strongly concentrate elements and particles present in the water column above. The higher accumulation rate of deep-sea sediments (millimetre per thousand years) results in a better time resolution but requires much larger sample volumes. With regard to other potential 244 Pu sources, we note that natural 244 Pu production on Earth is negligible and the ESS abundance has decayed to 10 −17 of its pre-solar value [22] , [23] . Anthropogenic production from atmospheric nuclear bomb tests and from high-power reactors is restricted to the last few decades, localized in upper layers and can easily be monitored through the characteristic isotopic fingerprint of the other co-produced 239–242 Pu isotopes. In fact the detection of anthropogenic 239,240 Pu in deep-sea sediments [38] , [39] , [40] and crusts [41] provides an excellent proxy for the ingestion efficiency of dust from the high atmosphere into these reservoirs, together with their chemical processing towards the final analyzed samples (Methods). Selected terrestrial archives for extraterrestrial 244 Pu Terrestrial archives like deep-sea FeMn crust and sediment archives extend over the past tens of million years. Large dust grains entering Earth’s atmosphere have also been observed by radar detections [42] . Extraterrestrial dust particles, cosmogenic nuclides and terrestrial input sink to the ocean floor and are eventually incorporated into the FeMn crust or sediment. For actinide transport through the latter stages, the observed deposition of global fallout [41] from atmospheric nuclear bomb testing [38] , [39] in deep marine reservoirs after injection to the stratosphere serves as a proxy to extraterrestrial particles. We chose two independent archives: a large piece (1.9 and 0.4 kg samples) from a deep-sea manganese crust (237 KD from cruise VA13/2, collected in 1976) with a growth rate between 2.5 mm per My (refs 29 , 37 ) and 3.57 mm per My (ref. 43 ). It originates from the equatorial Pacific (location 9°180′N, 146°030′W) at a depth of 4,830 m and covers the last ~25 My (refs 30 , 43 , 44 , 45 ). In the very same crust, the live 60 Fe signal mentioned above was found at about 2.2 My before present (BP) [28] , [29] . Our second sample, also from the Pacific Ocean, is a piston-core deep-sea sediment (7P), extracted during the TRIPOD expedition as part of the Deep-Sea Drilling Project (DSDP) at location 17°30′ N, 113°00′ W at 3,763 m water depth and covers a time period of ~0.5–2.1 My BP (W. Smith, Scripps Geological Collections, USA, personal communication). 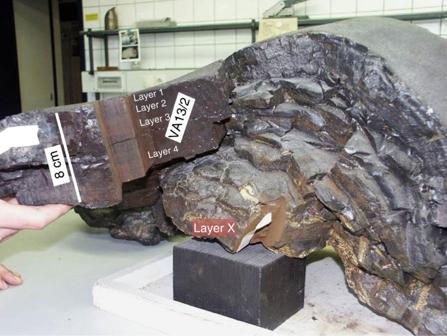Figure 1: Crust sample 237 KD. This FeMn crust (with a total thickness of 25 cm) was sampled in 1976 from the Pacific Ocean at 4,830 m water depth: large samples used in this work were taken from one part of the crust (hydrogenous crust, layers 1–4, left in the figure)) and from the bottom (hydrothermal origin, layer X, crust started to grow ~65 My ago43, see also refs44,45). The crust sample, covering a total area of 227.5 cm 2 and a time range of 25 My, was split into four layers (1–4) representing different time periods in the past (see Table 1 ). Each layer was subdivided into three vertical sections (B, C and D) with areas between 70 and 85 cm 2 , totalling 12 individually processed samples. The surface layer (layer 1, with a time range from present to 500,000 years BP) contains also the anthropogenic Pu signal originating from global fallout of atmospheric weapons testing [38] , [39] . Next, layer 2 spans a time period from 0.5–5 My BP, layer 3 5–12 My and layer 4 12–25 My (ref. 30 ). We note, the age for samples older than 14 My, where no 10 Be dating is possible [29] , [37] , is more difficult to establish; different age models suggest a time period of 12 to ~18–20 My (ref. 44 ), another model up to ~30 My (ref. 45 ) for layer 4). Finally, sample X, the bottom layer of hydrothermal origin ( Fig. 1 ) served as background sample. Table 1 244 Pu detector events and corresponding ISM flux compared with galactic chemical models assuming steady state. Full size table Figure 1: Crust sample 237 KD. This FeMn crust (with a total thickness of 25 cm) was sampled in 1976 from the Pacific Ocean at 4,830 m water depth: large samples used in this work were taken from one part of the crust (hydrogenous crust, layers 1–4, left in the figure)) and from the bottom (hydrothermal origin, layer X, crust started to grow ~65 My ago [43] , see also refs 44 , 45 ). Full size image For archives accumulating millions of years, the expected 244 Pu abundance range (see discussion) is well within reach of accelerator mass spectrometry (AMS), an ultra-sensitive method [46] , [47] , [48] of ion identification and detection. Based on the ingestion efficiency of Pu into deep-sea manganese crusts (21%) and on the AMS 244 Pu-detection efficiency (1 × 10 −4 , see Methods), we calculate a measurement sensitivity expressed as a 244 Pu flux onto Earth of the order of 0.1 to 1 atom per cm 2 per My 244 Pu from ISM deposition. Thus, for the crust with a 25 My accumulation period and with 200 cm 2 surface area ~500–4,000 244 Pu-detection events are expected, and about a factor 100 less for the sediment sample (1.64 My time period and 4.9 cm 2 surface area). 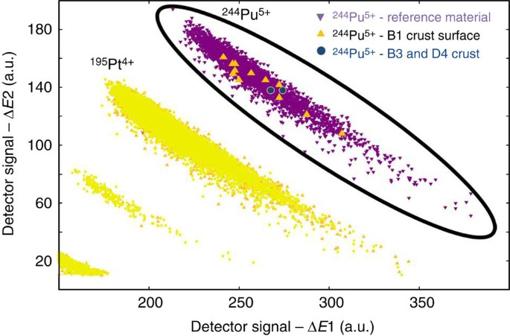Figure 2:244Pu detection with AMS. Identification spectra obtained in the AMS measurements with a particle detector (two independent differential energy-loss signals (ΔE1 and ΔE2) are plotted inx- andy-axis). Parasitic (or background) particles of different energy (for example,195Pt4+) and different mass were clearly separated and do not interfere. Displayed is an overlay of244Pu5+events obtained in a series of measurements for a244Pu reference material (purple triangle), the 12 events registered for one of the surface layer samples, B1 (yellow triangle) and the 2 events measured for the deeper layers B3 and D4, respectively (blue circle). Table 2 Expected 244 Pu fluxes at 1 AU from models and satellite data. Full size table AMS experimental data of 244 Pu abundances in Earth archives We have developed the capability to detect trace amounts of 244 Pu in terrestrial archives by AMS [46] and our technique provides background-free 244 Pu detection with an overall efficiency (atoms detected/atoms in the sample) of ~1 × 10 −4 (see Methods and Supplementary Tables 1–4 ). The AMS measurements determine the atom ratio 244 Pu/ A Pu where A Pu (A=236 or 242) is a spike of known amount (added during the chemical processing of the sample) from which the number of 244 Pu nuclei in the sample is obtained (see Methods). In addition to 244 Pu counting, we also measured the shorter lived 239 Pu ( t 1/2 =24.1 ky) content as an indicator of anthropogenic Pu signature. 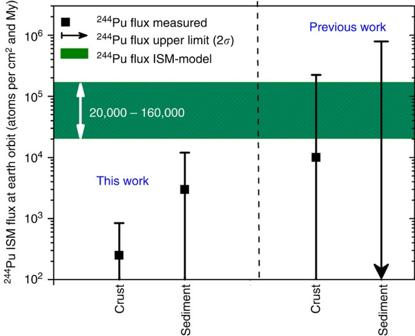Figure 3: Comparison of the measured244Pu flux at Earth orbit with models. The ISM244Pu flux at Earth orbit was determined from the concentrations measured in a deep-sea crust and a deep-sea sediment sample (note the logarithmic scale). Our results are compared with previous measurements (deep-sea crust41and sediment40) and to models of galactic chemical evolution18,50assuming steady-state conditions and taking into account filtration of dust particles when entering the heliosphere31. The arrows and error bars represent upper levels (2σ, 95% confidence levels) from the measurements. The green area indicates the data range deduced from the steady-state models. The crust data suggest a244Pu flux, which is a factor between 80 and 640 lower than inferred from the models. Table 3 Anthropogenic Pu at the surface and the incorporation efficiency into the manganese crust. Full size table The results for the four crust layers and the blank sample, obtained from the AMS measurements on 11 individual crust samples, are listed in Tables 1 and 3 (see also Supplementary Tables 1 and 2 ; identification spectra are plotted in Fig. 2 ). We observed one single event in each of the two crust subsamples, namely layer 3, section B (B3), and layer 4, section D (D4). No 244 Pu was registered in the other seven crust subsamples or the blank sample (X). A clear anthropogenic 239 Pu and 244 Pu signal, originating from atmospheric atomic-bomb tests from ~1950 to 1963, was observed in the top layer (16 events of 244 Pu detected). Measurements of samples from deep layers (>0.5 My) show also some events during the 239 Pu measurement (compared with the top layer, the 239 Pu count rate in the deep crust layers were a factor of ~100 lower, and the one in the sediment and blank sample were a factor of ~1,000 lower). Since naturally produced 239 Pu in these older layers is considered negligible, its presence is attributed to 238 U still present in the final AMS sample at about 8 to 9 orders of magnitude higher than 239 Pu and mimicking 239 Pu detector events (see Methods); we also note that the 236 Pu spike added for tracing the measurement efficiency was found to contain some 239 Pu, which we corrected for, see Supplementary Table 4 ). We conclude from the 239 Pu data that anthropogenic contamination did not add any significant 244 Pu detector events for all older layers (using the anthropogenic 244 Pu/ 239 Pu ratio obtained from the top layer, 1 × 10 −4 , see Methods, Table 3 ). In the following, we calculate for all cases 2 σ upper limits, that is, 95% confidence levels for which 0 (1 or 2) 244 Pu events corresponds to an upper limit of <3 (5 or 6.7, respectively) 244 Pu events (applying statistics for small signals [49] ). Figure 2: 244 Pu detection with AMS. Identification spectra obtained in the AMS measurements with a particle detector (two independent differential energy-loss signals (Δ E 1 and Δ E 2) are plotted in x - and y -axis). Parasitic (or background) particles of different energy (for example, 195 Pt 4+ ) and different mass were clearly separated and do not interfere. Displayed is an overlay of 244 Pu 5+ events obtained in a series of measurements for a 244 Pu reference material (purple triangle), the 12 events registered for one of the surface layer samples, B1 (yellow triangle) and the 2 events measured for the deeper layers B3 and D4, respectively (blue circle). Full size image 244 Pu flux deduced from measured terrestrial concentrations The crust data for all sections and for all three deeper layers are compatible (for details see also Supplementary Table 1 ). Owing to a higher chemical yield (integral sensitivity, column 5, Table 1 ) layers 3 and 4 provide lower limits. The measured 244 Pu concentration in these layers can be converted into a 244 Pu particle flux using chemical yield, detection efficiency, the incorporation efficiency of Pu into the crust (21±5 %, see Methods and Table 3 ), and the area and time period covered. We also assume that the extraterrestrial 244 Pu flux through Earth’s cross-section is homogeneously distributed over the Earth’s surface. Hence, the interstellar flux is calculated by multiplying the measured flux into the crust by a factor of 4/0.21=19. We thus derive a 2σ limit [49] for the 244 Pu-ISM-flux at Earth orbit from data of the three layers <3,500, <1,300 and <1,560 244 Pu atoms per cm 2 per My, and the one 244 Pu event in layers 3 and 4 corresponds to a flux of 247 +1,000 −235 and 320 +1,250 −300 atoms cm −2 per My, respectively. Combining all samples (2 244 Pu events) a flux of 250 +590 −205 and a 2σ-limit on the 244 Pu flux of <840 244 Pu atoms per cm 2 per My is obtained. The data are plotted in Fig. 2 . The single 244 Pu event measured for the deep-sea sediment converts to a flux of 3,000 (<15,000) atoms per cm 2 per My. Both archives give consistent 244 Pu flux limits with a higher sensitivity for the crust samples. First, we estimate the expected 244 Pu flux from ISM dust particles penetrating the SS, and their incorporation into terrestrial archives. Our experimental results are then compared with these estimations. Based on a uniform production model [18] or an open-box model [5] , [16] , [50] (see also ref. 24 ), taking into account Galactic-disk enrichment in low-metallicity gas, the present-day ISM atom ratio 244 Pu/ 238 U from SN events is calculated to be between 0.017 and 0.044 ( Table 2 ). We further assume that the abundance of 238 U in ISM dust is the same as that of chondrite meteorites [51] (corrected for the SS age), 1.7 × 10 −8 g per g meteorite, and derive a steady-state 244 Pu abundance of (2.8–7.5) × 10 –10 g Pu per g ISM (that is, (0.8–2.2) × 10 −14 atoms per cm 3 ); similar values are obtained if normalized to 232 Th. For interstellar dust particles (ISDs) entering the SS [27] , we have to take into account filtering when penetrating the heliosphere. ISDs were observed by the Ulysses, Galileo and Cassini [31] , [52] space missions over more than 5 years, for distances from the Sun between 0.4 and >5 AU. Measurements of the Cassini space mission [27] , [31] determine a mean flux of ISM dust of (3–4) × 10 −5 particles per m 2 per s at a distance of 1 AU, that is, at Earth’s position, with a mean particle mass of (3–7) × 10 −13 g (0.5–0.6 μm average particle size). These particles show a speed distribution corresponding to the flow velocity of the ISM (26 km s −1 ) and constitute 3–9% of the dust component of the ISM intercepted by the SS (see Table 2 ). The direct collection of a few particles identified as ISD, very recently reported [53] , although of low statistical significance, supports the scenario of penetration of large ISD particles into the inner SS and may be consistent with the satellite data. It should be noted that Galactic cosmic-rays penetrate the SS and recent observations clearly demonstrate therein the presence of Th and U, and tentatively of 244 Pu (ref. 54 ). Within the assumptions described above, the expected flux of 244 Pu atoms from the ISM reaching the inner SS (at Earth orbit) is (2.5–21) × 10 −31 g Pu per cm 2 per My or 20,000–160,000 244 Pu atoms per cm 2 per My. If evenly distributed over the Earth’s surface (that is, assuming a unidirectional ISM flux) the 244 Pu flux into terrestrial archives becomes 5,000–40,000 244 Pu atoms per cm 2 per My. Our experimental results ( Table 1 ) provide for the first time a sensitive limit of interstellar 244 Pu concentrations reaching Earth, integrated over a period of 24.5 My. Our data are a factor of 80–640 lower than the values expected under our constraints on ISM grain composition from a SN derived steady-state actinide production (the 2 σ upper limit of ~840 atoms per cm 2 per My is still a factor of 25–200 lower). The lifetime of 244 Pu is comparable to the complete mixing time scales of the ISM [32] , [33] , [34] . The deep-sea crust sample integrates a 244 Pu flux over a time period of 24.5 My (~1/10 of the SS rotation period in the Galaxy) corresponding to a relative travel distance of the SS of 650 pc (taking the mean speed of the measured ISM dust particles of 26 km s −1 (ref. 52 ), ~1/10 of the galactic orbital speed, as a proxy for ISM reshaping and for motion differences relative to the co-rotating local neighbourhood). These results, consistent with previous studies on extraterrestrial 244 Pu in crust [41] , [55] and sediment samples [40] , [56] , are more sensitive by a factor of >100 and provide for the first time stringent experimental constraints on actinide nucleosynthesis in the last few hundred million years (see Fig. 3 ). Figure 3: Comparison of the measured 244 Pu flux at Earth orbit with models. The ISM 244 Pu flux at Earth orbit was determined from the concentrations measured in a deep-sea crust and a deep-sea sediment sample (note the logarithmic scale). Our results are compared with previous measurements (deep-sea crust [41] and sediment [40] ) and to models of galactic chemical evolution [18] , [50] assuming steady-state conditions and taking into account filtration of dust particles when entering the heliosphere [31] . The arrows and error bars represent upper levels (2 σ , 95% confidence levels) from the measurements. The green area indicates the data range deduced from the steady-state models. The crust data suggest a 244 Pu flux, which is a factor between 80 and 640 lower than inferred from the models. Full size image A simple steady-state scenario might represent a simplified assumption within our local ISM environment. Compared with the typical size of ISM substructures of ~50–100 pc (for example, LB) [27] , [32] , [33] , [34] , [57] and life-times of some 10 My, the crust sample probes, however, the equivalent of ~10 such cavities (the 244 Pu life-time coupled with the spatial movement of the SS during the 24.5 My accumulation). Thus, we expect existing ISM inhomogeneities largely smeared out in our space- and time-integrated samples, confirming the significance of a ratio <1/100 between measured and expected 244 Pu abundance. Further, we can relate our result to actinide nucleosynthesis during the recent SN history of the LB [32] , [33] , [34] , [58] , [59] in which the SS is embedded now. ISM simulations suggest the LB was formed by ~14–20 SN explosions within the last 14 My (refs 32 , 33 , 34 ) with the last one ~0.5 My BP (refs 32 , 58 ). To reproduce size and age of the LB, an intermediate density of seven particles per cm 3 (~10 times the mean density of the local environment now) before the first SN explosion took place, is required [34] . The mean mass density of the LB has since transformed to 0.005 particles per cm 3 . The series of SNe explosions has generated the void inside the LB and has continuously pushed material into space forming an ISM shell. The SS is now placed inside the LB and thus has passed or passes the front of accumulated swept-up material including possible pre-existing 244 Pu from nucleosynthesis events prior to the formation of the LB [35] , [36] . We can distinguish three different scenarios for the recent LB history: (i) the SN activity transformed the local ISM from a dense to a low-density medium (LB), and pre-existing ISM material containing (steady state) old 244 Pu was swept-up and passed the SS [35] , [60] ; (ii) direct production of 244 Pu in the 14–20 SNe and their expected traces left on Earth [35] ; and (iii) independently, we can compare our data for 244 Pu with recent AMS data of 60 Fe influx [28] , [29] . In a simple first order estimate for scenario (i), we assume that the swept-up material is distributed over a surface with a radius of 75 pc. Using the pre-LB density of seven particles per cm 3 (ref. 34 ) with 1% of this ISM mass locked into dust, we calculate with our assumptions of Pu concentration in dust ( Table 2 ) and a dust penetration efficiency of ~6±3% into the SS to Earth orbit, a 244 Pu fluence from swept-up material of (0.4–3) × 10 6 244 Pu atoms per cm 2 (see Table 2 ). Our experimental data give a flux of 200 +800 −200 244 Pu atoms per cm 2 per My for the last 12 My (layers 2 and 3) at Earth orbit corresponding to a fluence of 2,300 (<12,000) 244 Pu atoms per cm 2 during this period. This experimental value for the fluence is a factor of ~170–1,300 lower than the value calculated above (see Table 2 ) assuming swept-up material of about half the diameter of the LB is moved across the SS. We deduce approximately the same discrepancy as found for a simple steady-state actinide production scenario. For LB scenario (ii), in a first order estimation, we take the SN-rate of 1.1–1.7 SNe/My within the LB [34] , [58] and a mean distance to the SS for these SN events of 100 pc. From our measured value of 200 +800 −200 244 Pu atoms per cm 2 per My at Earth orbit (with 6% penetration efficiency into 1 AU), this corresponds to ~3,000 (<17,000) 244 Pu atoms per cm 2 per My unfiltered ISM flux, spread over a surface area with a radius of 100 pc. We deduce an average 244 Pu yield per SN of (0.6 +2.4 −0.6 ) × 10 −9 M solar for the last 12 My. Finally for LB scenario (iii), Knie et al . [28] and Fitoussi et al . [29] measured a clear 60 Fe signal of possible SN origin ~2.2 My in the past in exactly the same crust material (237 KD) as we have used in this work for the search of 244 Pu (using a sample ~50 cm distant; a SN origin for 60 Fe is being questioned by some authors [61] , [62] , while several recent studies on 60 Fe in deep ocean sediments [63] , [64] and in lunar samples [65] confirm the results of Knie et al . [28] ). Thus we can directly compare the measured fluences of 60 Fe and 244 Pu for the same event (using layer 2, 0.5–5 My). These fluence values can be converted into an atom ratio that is independent of the SS penetration efficiency and we assume the same incorporation efficiency for Fe and Pu (refs 63 , 64 , 65 , 66 ). We deduce a 244 Pu/ 60 Fe isotope ratio for this event of <6 × 10 −5 (similarly, we obtain an upper limit from the sediment of <10 −4 ). Clearly, this ratio depends strongly on the type of explosive scenario. Literature values for this ratio are highly varying also due to large uncertainties in the r -process yields. Our experimental results indicate that SNe, at their standard rate of ~1 to 2 per 100 years in the Galaxy, did not contribute significantly to actinide nucleosynthesis for the past few hundred million years and actinide nucleosynthesis, as mapped through live 244 Pu, seems to be very rare. Our data may be consistent with a predominant contribution of compact-object mergers, which are 10 2 to 10 3 less frequent than core-collapse SNe [1] . A recent observation indicates indeed that such mergers may be sites of significant production of heavy r -process elements [10] , [11] . Our experimental work is also in line with observations of low-metallicity stars [12] , [14] , indicating splitting into a rare and a more frequent r -process scenario allowing an independent evolution of the r -process elements Eu/Th over time [3] , [4] . In addition, we must conclude from our findings that, given the presence of short-lived actinide 244 Pu (and 247 Cm) in the ESS, it must have been subject to a rare heavy r -process nucleosynthesis event shortly before formation. Details on the chemistry of the crust samples Quantitative extraction of Pu was required from the 2.3 kg crust sample. The sample potentially contained some 10 6 –10 7 atoms of 244 Pu, which correspond to an atom-concentration of (0.5–5) × 10 −19 relative to the bulk material. No stable isobar to 244 Pu exists in nature and molecular interference in the measurements is excluded. The FeMn crust sample was split into four layers 1–4 and three sections B, C and D. The top layer (1 mm, ‘crust modern’) was removed for measuring the anthropogenic Pu content originating from atmospheric atomic-bomb tests from ~1950 to 1963. Four different vertical layers represent different time periods in the past, while three different horizontal sections were chosen to identify possible lateral variations (B, C and D). The 12 individual pieces had masses between 30 and 360 g. Ten samples were measured by AMS. The individual parts of the crust were dissolved in aqua regia and H 2 O 2 , and a spike of ~3 × 10 8 atoms of a 236 Pu reference material was added to the leached solutions. After removal of the undissolved SiO 2 fractions, the solutions were brought to dryness and successively redissolved in concentrated HNO 3 and H 2 O 2 . At this stage, the sample solutions contain the actinides, but also the dominant fraction of the matrix elements of the crust, in particular Mn (~14 to 28%) and Fe (~16 to 28%). To separate the actinides from the Mn and Fe fraction, a pre-concentration step involving the selective co-precipitation of the actinides with CaC 2 O 4 at pH ~1.7 was performed. After centrifugation, the precipitated CaC 2 O 4 was converted to CaCO 3 in a muffle furnace at a temperature of 450 °C for several days. The CaCO 3 was dissolved in 7.2 M HNO 3 and the oxidation state of Pu was adjusted quantitatively to (IV)Pu by the addition of NaNO 2 . These solutions were then loaded onto pre-conditioned anion-exchange columns containing Dowex 1 × 8, from which after the separation of the Ca, Am, Cm and the Th fractions Pu was eluted by reduction to (III)Pu with a solution of HI. To purify the obtained Pu fraction, two additional successive anion-exchange separations similar to the one described above were performed on the eluted Pu solutions. The Pu fractions were further purified from the organic residues by fuming with HNO 3 and H 2 O 2 . Successively an Fe(OH) 3 co-precipitation of Pu was performed in 1 M HCl by adding 2 mg of Fe powder. After centrifugation and drying of the precipitate, the Fe(OH) 3 was converted to iron oxide by combustion in a muffle furnace at 800 °C for 4 h. The plutonium oxide embedded in a matrix of iron oxide was then mixed with 2 mg of high-purity Ag powder and pressed in the sample holders suitable for the subsequent AMS measurement. Owing to the massive matrix component of the crust for some samples a low chemical yield was observed (in the AMS measurements via the 236 Pu spike). In these cases the procedure for Pu extraction was repeated, that is, the solutions containing the Mn and Fe fraction underwent again a CaC 2 O 4 co-precipitation procedure and the resulting actinide fractions were mixed with the rest of the remaining fractions originating from the first threefold anion-exchange separation. These solutions underwent a chromatographic column separation employing Tru-resin in 5 M HCl, from which after the elution of the Ca, Am and Cm and the Th fractions Pu was stripped out with a solution of 0.03 M H 2 C 2 O 4 in 0.5 M HCl. Chemical processing of the TRIP deep-sea sediment Similarly, Pu was extracted from two deep-sea sediment samples of 43 and 58 g mass provided by the Scripps Oceanographic Institute, the University of California at San Diego. It was a piston core (7P), extracted during the TRIPOD expedition (1966) as part of the DSDP at location 17°30′ N 113°00′ W (Pacific Ocean) at 3,763 m water depth. Two main sections were sampled with sediment depths 0–80 cm and 80–230 cm, from which the top 3 cm (containing the anthropogenic Pu) were removed. One quarter of the total cross-section throughout the ~230 cm length of the core was used in this study (4.9 cm 2 ). The samples, shipped in sealed polyethylene, were chemically processed at the Hebrew University, Jerusalem. The physical and chemical processing of the sediments is as follows: the processing involved brief milling and calcination of the sample, alkali fusion of the sediment using NaOH at 750 °C, liquid-phase extraction of Fe and other main elements and liquid ion-chromatography to extract the Pu fraction. Prior to the alkali fusion steps, an isotope 242 Pu marker and a chemical 230 Th marker were added to the sediment. 242 Pu was used to monitor the efficiency of Pu detection by measuring the 242 Pu content of the final AMS sample (analogous to the 236 Pu spike in the crust samples), while 230 Th served as additional indicator of the chemical efficiency of actinide extraction by measuring the alpha activity of an electroplated deposition prepared from a separate fraction. The final AMS samples were obtained by co-precipitation of the Pu fraction with Fe in an ammonia solution, centrifugation and ignition to obtain a Fe 2 O 3 matrix containing the Pu marker and traces. Finally, 2 mg of high-purity Ag powder was added and the powder pressed in the sample holders suitable for the subsequent AMS measurement. AMS-measurement procedure We have applied the most sensitive technique—AMS [46] , [47] , [48] to detect minute amounts of 244 Pu. This technique provides the complete suppression of any interfering background, for example, molecules of the same mass, by the stripping process in the terminal of a tandem accelerator, which is crucial for such experiments where only a few counts are expected. The 244 Pu measurements were performed at the Vienna Environmental Research Accelerator (VERA) facility in the University of Vienna [46] , [67] , [68] , [69] . This set up has been optimized for high-measurement efficiency and offered an exceptional selectivity. The individual crust samples were spiked with a well-known amount of 236 Pu atoms ( 242 Pu for the sediment). 244 Pu and 239 Pu measurements were performed relative to the 236 Pu ( 242 Pu) spike, that is, the total efficiency and the chemical yield of Pu (when compared with the theoretical measurement efficiency) were monitored with the 236 Pu ( 242 Pu) spike, that was counted in short time intervals before and after the 244 Pu runs in the AMS measurements. The chemical yield varied between 5 and 70% largely depending on the sample matrix. In a sputter source, the Fe/Ag matrix, containing the Pu atoms, was bombarded with Cs ions and negative PuO ions were extracted, and energy and mass were analyzed before injection into the tandem accelerator. The negative ions were accelerated to the 3 MV tandem terminal and stripped there to positive ions in the gas stripper (O 2 ). 244 Pu 5+ ions were accelerated to a final energy of 18 MeV and selected with a second analyzing magnet. They then had to pass an additional energy and another mass filter (electrostatic and magnetic dipoles, respectively) and were finally counted in an energy-sensitive particle detector. The system was optimized with a 238 U pilot beam and monitored during a measurement with reference samples containing 242 Pu. The measurement set up for 244 Pu and 236 Pu counting was scaled from the tuning set up. At the end of a measurement series, reference samples containing a well-known isotope ratio of 244 Pu/ 242 Pu were measured. The measured ratios reproduced the nominal values within 4% and confirmed the validity of scaling between the different masses in the measurement. This set up suppresses adjacent masses (for example, 238 U from 239 Pu) by 8–9 orders of magnitude. This suppression factor was sufficient for 244 Pu counting as no interference from neighbouring masses is expected for 244 Pu (and additional isotopic suppression, for example, via time-of-flight identification, would have been at the cost of lower particle transmission). However, 238 U was abundant at levels of ~10 p.p.m. in the crust, and U separation from Pu in the chemical preparation of these samples was not 100%. Thus, the detector events registered for 239 Pu counting, by 2–3 orders of magnitude lower compared with modern samples, are attributed to leaking 238 U atoms injected as 238 UOH − ions together with 239 PuO − mimicking 239 Pu. To summarize, our detector event rate for 239 Pu suggests no significant anthropogenic 244 Pu contamination. The measurement procedure was a sequence of alternating counting periods of 236 Pu, 239 Pu, 244 Pu and again 236 Pu. All samples were repeatedly measured until they were completely exhausted. The sputtering time per sample was between 5 and 20 h. Three measurement series were required to fully consume all the samples. The overall yields for the 12 crust samples were between 0.06 × 10 −4 and 1.54 × 10 −4 , that is, one 244 Pu detector event would represent correspondingly between 6,500 and 1.7 × 10 5 244 Pu atoms in the analyzed sample. A similar procedure was followed for the sediment samples where 242 Pu was used as a spike. Due to the low number of expected detector events, the machine and measurement backgrounds were carefully monitored with samples of pure Fe and Ag powders. They were sputtered identical to the samples containing the crust fractions. In addition, one crust sample (X), the lowest layer of the crust material, was of hydrothermal origin where no extraterrestrial 244 Pu could accumulate. This sample was chemically prepared and measured in the same way as the other crust samples and served as a process blank for potential chemistry and machine background. Incorporation efficiency of Pu into the deep-sea crust The incorporation efficiency of bomb-produced Pu into the crust was determined from the anthropogenic 239 Pu content in the top layer of the crust and deep-sea sediment data (details are given in Table 3 ). The total measurement efficiency is calculated from the total number of 236 Pu registered and normalized by the time fraction of 236 Pu AMS counting and divided by the number of 236 Pu atoms added as spike to the sample (3 × 10 8 atoms each). The number of 244 Pu atoms per sample is calculated from the number of 244 Pu events registered with the particle detector, scaled by the time fraction of AMS 244 Pu counting time and normalized with the measurement efficiency; the same procedure was used for 239 Pu atoms per sample. The 239 Pu detector events were corrected for a well-known contribution when adding the 236 Pu spike, which also contains 239 Pu (see Supplementary Table 1 for more details). The average over 18 sediment cores from the Pacific measured between 1974 and 1979 gave a 239,240 Pu sediment inventory of 2.15 Bq m −2 (ref. 38 ). When compared with the well-known surface activity of 2.8 mCi km −2 (104 Bq m −2 ) [39] , at the time of sampling the crust in 1976, 2.1% of anthropogenic Pu from the bomb tests was incorporated into deep-sea sediments with sediments having an incorporation efficiency of 100% (this compares well with the ratio of the time that had passed since the peak in atmospheric bomb-testing (15 years) and the mean residence time of Pu in the ocean of ~440 years; this ratio is, 3.4%). Taking the total anthropogenic Pu-inventory at the location of the crust (between 60 and 78 Bq m −2 and a 240 Pu/ 239 Pu atom ratio of 0.20; refs 40 , 41 ); and the fraction of 2.1% measured in sediments, we found that 8.2 × 10 7 239 Pu atoms per cm 2 have reached the crust in the year 1976. We measured from the three crust subsamples from the top layer a 239 Pu surface density of (1.76±0.44) × 10 7 cm −2 , and thus deduce an incorporation efficiency into the crust of (21±5)%. We assume that the ISM-Pu is incorporated like the bomb-produced Pu. How to cite this article: Wallner, A. et al . Abundance of live 244 Pu in deep-sea reservoirs on Earth points to rarity of actinide nucleosynthesis. Nat. Commun. 6:5956 doi: 10.1038/ncomms6956 (2015).